Anex vivogene therapy approach to treat muscular dystrophy using inducible pluripotent stem cells Duchenne muscular dystrophy is a progressive and incurable neuromuscular disease caused by genetic and biochemical defects of the dystrophin–glycoprotein complex. Here we show the regenerative potential of myogenic progenitors derived from corrected dystrophic induced pluripotent stem cells generated from fibroblasts of mice lacking both dystrophin and utrophin. We correct the phenotype of dystrophic induced pluripotent stem cells using a Sleeping Beauty transposon system carrying the micro-utrophin gene, differentiate these cells into skeletal muscle progenitors and transplant them back into dystrophic mice. Engrafted muscles displayed large numbers of micro-utrophin-positive myofibers, with biochemically restored dystrophin–glycoprotein complex and improved contractile strength. The transplanted cells seed the satellite cell compartment, responded properly to injury and exhibit neuromuscular synapses. We also detect muscle engraftment after systemic delivery of these corrected progenitors. These results represent an important advance towards the future treatment of muscular dystrophies using genetically corrected autologous induced pluripotent stem cells. Pluripotent stem cells are particularly attractive for therapeutic application as these cells are endowed with robust expansion potential, enabling the generation of large quantities of tissue-specific stem/progenitor cell preparations. This is extremely beneficial as cell number has been one of the main barriers to implementing cell-based therapies. Induced pluripotent stem (iPS) technology [1] , [2] , [3] , [4] further allows for the derivation of patient-specific pluripotent stem cell preparations without the ethical and immunological concerns associated with human embryonic stem (ES) cells. In the case of muscular dystrophies, either allogeneic or autologous cell transplantations have the potential to lead to an effective treatment. For allogeneic transplantation, one would utilize iPS-derived myogenic progenitors obtained from a healthy HLA-matched donor, which following transplantation would give rise to new healthy myofibers, as well as fuse to the recipient’s myofibers, to generate hybrid myofibers that express dystrophin. The autologous approach would require ex vivo genetic correction of dystrophic iPS cells before transplantation. Despite extensive research in iPS technology, to date there are only two reports on the therapeutic potential of disease-specific iPS cells that have been genetically corrected, transplanted back into an appropriate mouse model and shown to provide therapeutic benefit: for sickle cell anaemia [5] and β-thalassaemia [6] . Genetic correction for muscular dystrophies has been tested with some success in mesoangioblasts [7] , [8] , [9] ; however, these somatic cells have reported limited expansion potential [10] . The deficit in translational studies involving genetically corrected iPS cells is most likely because of the difficulty in coaxing pluripotent stem cells to become lineage-specific stem cells that are able to produce functional tissue in vivo . We developed and continued to improve a method to efficiently generate skeletal muscle stem/progenitor cells endowed with significant regeneration potential through Pax3 or Pax7 induction in control ES and iPS cells [11] , [12] , [13] , [14] . In the present study, we show proof-of-principle for the ex vivo gene correction of mouse dystrophic iPS cells. We inserted the micro-utrophin (μUTRN) gene into iPS cells obtained from dystrophin/utrophin double knockout (dKO) mice using the Sleeping Beauty transposon (Tn) system, and demonstrated that skeletal myogenic progenitors derived from gene-corrected iPS cells have the capacity to promote substantial muscle regeneration in vivo when transplanted back in dKO mice, and that engraftment is accompanied by functional improvement. Characterization and correction of dystrophic iPS cells To address the feasibility of using disease-specific iPS cells and genetic correction in the context of Duchenne muscular dystrophy (DMD), we utilized the dystrophin/utrophin dKO mouse model as the source of tail-tip fibroblasts (TTFs), as well as recipients of iPS-derived therapeutic myogenic cell preparations ( Fig. 1a ). This choice was based on the fact that mdx mice, although a favourite model for DMD [15] , present a mild phenotype, attributed to compensatory overexpression of the dystrophin-related protein, utrophin [16] . The dKO mice, which lack both dystrophin and utrophin, present a severe phenotype characterized by progressive muscle wasting, impaired mobility, abnormal breathing pattern, cardiomyopathy and premature death [17] , [18] , which more closely resembles DMD in human patients. To restore the dystrophin-glycoprotein complex (DGC), we chose to re-express a μUTRN transgene, which has been shown to ameliorate the dystrophic phenotype [19] , [20] , [21] , [22] . This approach tests a vector that would potentially be preferred in human patients because it would avoid the immune response that is elicited by the dystrophin-naive immune system (the mouse model tests function of μUTRN in this context, but not immune aspects). As summarized in Fig.1a , the therapeutic strategy applied in the present study involved (1) reprogramming of dystrophic donor fibroblasts into iPS clones, (2) genetic repair of selected iPS clones with μUTRN using the non-viral Sleeping Beauty Transposon (Tn) System, (3) in vitro differentiation of corrected iPS cell clones into myogenic progenitors and (4) transplantation of corrected myogenic precursors into dystrophic dKO mice (mdx; utrn −/− ). 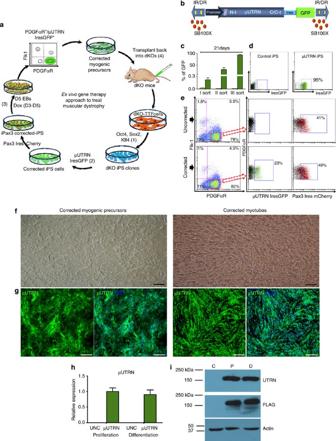Figure 1:Ex vivocorrection of dystrophic iPS cells. (a) Scheme of theex vivogene therapy approach, which involves (1) reprogramming of dystrophic donor-derived fibroblasts into iPS cells, (2) genetic repair of iPS cells with the μUTRN transgene using theSleeping BeautyTn system, (3) generation of myogenic progenitors from corrected iPS cells through Pax3 induction and (4) transplantation of corrected myogenic precursors into dystrophic donor mice. (b) TheSleeping BeautyTn system: the Tn contains the hEF1α-eIF4g promoter, the μUTRN gene and an iresGFP. The whole transgene is flanked by the terminal inverted repeats (IR/DR, arrowheads), each containing two binding sites for the transposase (DR, yellow arrows). The transposase protein SB100X (red spheres) catalyses integration of the Tn into the genome with high efficiency. (c) Left panel: Graphic bars represent percentage of GFP+cells obtained before each sorting. Green bars correspond to iPS cells nucleofected with pKT2/μUTRN-iresGFP/SB100X, whereas yellow bars represent controls, iPS cells transduced with pKT2/μUTRN-IresGFP only (no transposase). Data are mean±s.e.m. of three independent samples. (d) FACS profile for GFP shows stable expression of μUTRN in corrected iPS cells (right panel), whereas control iPS cells are GFP-(left panel). (e) Flow-cytometric analyses for Flk-1 and PDGFαR expression on day 5 EBs of Pax3-induced uncorrected (upper panel) and corrected iPS (lower panel) cells. The PDGFαR+Flk-1−cell fraction was gated (red square on left panels) and analysed for the expression of GFP, representing μUTRN+cells (middle panels), and mCherry, representing Pax3+cells (right panels). (f) Phase-contrast images of monolayers under proliferation (left) and differentiation (right) culture conditions. (g) Immunofluorescence staining for μUTRN (green) in proliferating iPS-derived myogenic progenitors (left) and their derivative myotubes (right). Cells are co-stained with 4,6-diamidino-2-phenylindole (DAPI) (blue). Scale bar, 200 μm. (h) Quantitative PCR analyses indicate relative expression of μUTRN in corrected iPS-derived myogenic cells under proliferation (P) and differentiation (D) conditions. Actin was used as house-keeping gene. UNC: uncorrected cells. Error bars represent s.e.m. from three replicates of three independent experiments. (i) Immunoblotting with anti-UTRN and anti-FLAG antibodies confirms the presence of 163 kDa μUTRN-only in corrected cells. Control uncorrected cells are labeled as C. Figure 1: Ex vivo correction of dystrophic iPS cells. ( a ) Scheme of the ex vivo gene therapy approach, which involves (1) reprogramming of dystrophic donor-derived fibroblasts into iPS cells, (2) genetic repair of iPS cells with the μUTRN transgene using the Sleeping Beauty Tn system, (3) generation of myogenic progenitors from corrected iPS cells through Pax3 induction and (4) transplantation of corrected myogenic precursors into dystrophic donor mice. ( b ) The Sleeping Beauty Tn system: the Tn contains the hEF1α-eIF4g promoter, the μUTRN gene and an iresGFP. The whole transgene is flanked by the terminal inverted repeats (IR/DR, arrowheads), each containing two binding sites for the transposase (DR, yellow arrows). The transposase protein SB100X (red spheres) catalyses integration of the Tn into the genome with high efficiency. ( c ) Left panel: Graphic bars represent percentage of GFP + cells obtained before each sorting. Green bars correspond to iPS cells nucleofected with pKT2/μUTRN-iresGFP/SB100X, whereas yellow bars represent controls, iPS cells transduced with pKT2/μUTRN-IresGFP only (no transposase). Data are mean±s.e.m. of three independent samples. ( d ) FACS profile for GFP shows stable expression of μUTRN in corrected iPS cells (right panel), whereas control iPS cells are GFP - (left panel). ( e ) Flow-cytometric analyses for Flk-1 and PDGFαR expression on day 5 EBs of Pax3-induced uncorrected (upper panel) and corrected iPS (lower panel) cells. The PDGFαR + Flk-1 − cell fraction was gated (red square on left panels) and analysed for the expression of GFP, representing μUTRN + cells (middle panels), and mCherry, representing Pax3 + cells (right panels). ( f ) Phase-contrast images of monolayers under proliferation (left) and differentiation (right) culture conditions. ( g ) Immunofluorescence staining for μUTRN (green) in proliferating iPS-derived myogenic progenitors (left) and their derivative myotubes (right). Cells are co-stained with 4,6-diamidino-2-phenylindole (DAPI) (blue). Scale bar, 200 μm. ( h ) Quantitative PCR analyses indicate relative expression of μUTRN in corrected iPS-derived myogenic cells under proliferation (P) and differentiation (D) conditions. Actin was used as house-keeping gene. UNC: uncorrected cells. Error bars represent s.e.m. from three replicates of three independent experiments. ( i ) Immunoblotting with anti-UTRN and anti-FLAG antibodies confirms the presence of 163 kDa μUTRN-only in corrected cells. Control uncorrected cells are labeled as C. Full size image Dystrophic iPS cells were generated by retroviral transduction of TTF cells using Oct4 , Klf-4 and Sox2 (ref. 23 ). iPS clones were initially screened by morphology, SSEA-1 expression and alkaline phosphatase activity ( Supplementary Fig. S1a,b ). Based on these markers, a subset of clones was selected for additional analysis, which included immunofluorescence staining to pluripotency markers ( Supplementary Fig. S1c ), as well as assessment of their ability to form embryonic mesoderm following in vitro differentiation into embryoid bodies (EBs), as evidenced by Flk-1 and PDGFαR expression ( Supplementary Fig. S1d–e ). After this analysis, one iPS clone (C3) was chosen for the studies presented here. These cells displayed normal karyotype and exhibited the ability to develop typical teratomas ( Supplementary Fig. S1f,g ). Importantly, following EB differentiation, iPS cells showed downregulation of pluripotency markers and normal expression of imprinted genes ( Supplementary Fig. S1h–i , respectively), which has been previously shown to distinguish fully reprogrammed iPS cells [24] . Dystrophic iPS cells were then corrected with the μUTRN transgene (R4-R21). This gene is a contracted version of UTRN-lacking sequences encoding spectrin-like repeats 4 through 21, but containing the N-terminal domain that binds to F-actin, and the C-terminal domain (C/C cysteine-rich domain) that interacts with the dystrophin–glycoprotein complex. This gene complements both the loss of dystrophin and utrophin [20] . The Sleeping Beauty Tn system has several advantages including efficient gene transfer and stable gene expression in mouse and human ES cells [25] , [26] , and reduced likelihood of insertional mutagenesis [27] . We developed a T2-inverted terminal repeat Tn vector (pKt2/μUTRN) carrying a 7.3-kb engineered transgene containing μUTRN and an iresGFP reporter ( Fig. 1b ), which allows for FACS selection of μUTRN-corrected iPS cells. SB100X ( Fig. 1b ) is a recently engineered hyperactive variant that yields high levels of Tn integration, leading to efficient and stable gene transfer [28] . We observed a stable gene-transfer frequency of 0.3%, 1 week after nucleofection with Tn and transposase vectors ( Fig. 1c ). Green fluorescent protein (GFP + ) cells were sorted, expanded and re-sorted, giving rise to a homogeneous and stable population of μUTRN-corrected iPS cells (>90% GFP + ) ( Fig. 1c , right panel). The expression of μUTRN was confirmed by quantitative PCR ( Supplementary Fig. S2a ). Corrected iPS cells maintained a normal karyotype ( Supplementary Fig. S2b ). Skeletal myogenic progenitors from gene-corrected iPS cells To enable the efficient generation of skeletal myogenic progenitors, both μUTRN-corrected and control (uncorrected) iPS cells ( Fig. 1d ) were modified to allow doxycycline-regulated conditional Pax3 expression, which we have previously shown allows the derivation of repopulating myogenic progenitors from ES cells [12] ( Supplementary Fig. S3a ). Pax3 + cells (mCherry + ) were detected only when dox was added to the culture medium ( Supplementary Fig. S3b ). This has been confirmed by western blot analysis ( Supplementary Fig. S3c ). To isolate skeletal myogenic precursors, Pax3 was induced from day 3 to day 5 of EB differentiation, at which point paraxial mesoderm progenitors were isolated based on the expression of PDGFαR and lack of Flk-1 ( Fig. 1e , left panels) [12] . In the case of corrected iPS-derived EBs, cells were further purified based on positivity for GFP, which is co-expressed with μUTRN ( Fig. 1e , lower middle panel). Because Pax3 is co-expressed with mCherry, both control and corrected dox-induced EBs were mCherry + ( Fig. 1e , right panels), whereas non-induced control counterparts were mCherry − ( Supplementary Fig. S3d ). PDGFαR + Flk-1 − GFP + -sorted cell preparations from corrected iPS-derived EBs ( Fig. 1e ) were expanded in the presence of basic fibroblast growth factor (bFGF) and doxycycline. Proliferating myogenic precursors emerged from these cultures ( Fig. 1f , left panels). When differentiation was induced in vitro , these had the ability to undergo final maturation, giving rise to multinucleated myotubes ( Fig. 1f , right panels) that exhibited elevated fusion index (82±8%; Supplementary Fig. S3e ) (details in methods). Importantly, abundant and stable expression of μUTRN was observed in corrected myogenic progenitors and their derivative myotubes, as shown by immunofluorescence staining ( Fig. 1g ), quantitative PCR ( Fig. 1h ) and western blot analysis ( Fig. 1i ). No utrophin was detected in control uncorrected myogenic preparations ( Fig. 1i ). As anticipated, proliferating myogenic progenitors were characterized by abundant expression of Pax3 as well as Myf5 ( Supplementary Fig. S4a ). Under these conditions, MyoD was observed in fewer nuclei, whereas terminal differentiation markers, such as MyHC, were barely detected ( Supplementary Fig. S4a ). This profile changed upon induction of myogenic differentiation, as multinucleated myotubes expressed high levels of MyHC and MyoD, and displayed significant downregulation of Pax3 and Myf5 ( Supplementary Fig. S4b ). These results were further confirmed by real-time RT–PCR ( Supplementary Fig. S5 ). Flow-cytometric analysis of μUTRN-corrected myogenic progenitors showed homogeneous expression of M-cadherin (99%), CD56 (82%), VCAM1 (85%), SYND-4 (98%) and CXCR4 (98%) ( Supplementary Fig. S4c ), surface markers characteristic of satellite and myogenic progenitor cells [29] . Regenerative potential of gene-corrected myogenic cells To assess whether these corrected autologous cells would engraft and differentiate into muscle in vivo , μUTRN-corrected iPS-derived myogenic precursors were transplanted into the left tibialis anterior (TA) muscles of 3-week-old dKO mice, whereas the contra-lateral TA (right) was injected with PBS. Because the dKO strain presents a much more severe phenotype, we did not pre-injure with cardiotoxin (CTX) to enhance engraftment, as previously described for transplantations in mdx mice [12] . Mice received immunosuppression daily (Tacrolimus) as both dystrophin and utrophin are foreign proteins to these mice, in addition to GFP. Three weeks following transplantation, cryosections of TA muscles were evaluated for engraftment by immunofluorescence staining for utrophin using a polyclonal antibody that specifically recognizes the amino-terminal epitope preserved in the μUTRN transgene. As expected [17] , [18] , no expression of utrophin was detected in PBS-injected control muscles of the contra-lateral leg ( Fig. 2a ). On the contrary, TA muscles that had been transplanted with μUTRN-corrected iPS-derived myogenic precursors demonstrated substantial engraftment, as showed by the clear expression of utrophin in recipient muscles ( Fig. 2b ). Quantification of μUTRN + myofibers showed engraftment average levels of 19±7.6% in transplanted mice ( Fig. 2c ). Analyses for β-dystroglycan, α1-syntrophin and neuronal nitric oxide synthase in consecutive sections revealed contiguous expression of these proteins across long sections of engrafted μUTRN + myofibers ( Fig. 2b ). These data show that μUTRN-corrected iPS-derived myogenic precursors are able to engraft in vivo , and, more importantly, μUTRN expression was able to restore other components of the DGC, which are missing in the absence of dystrophin ( Fig. 2a ) [17] , [18] , [30] , [31] . Another critical aspect is that no tumour was detected in any of the transplanted mice (total of 20 dKO mice) or in NOD/SCID mice injected with these cell preparations up to 3 months post transplantation. We have previously shown that by incorporating positive selection for paraxial mesoderm markers, teratoma-forming cells can be eliminated from mouse ES-derived cell preparations [12] . 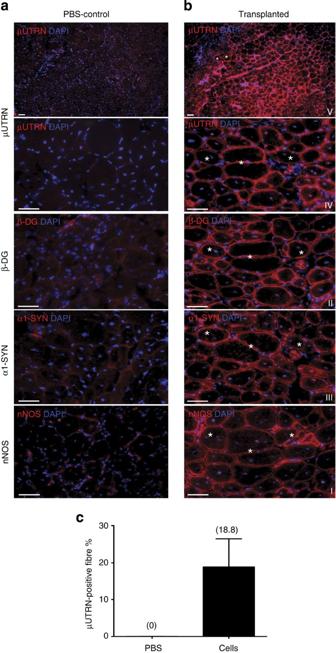Figure 2: Engraftment of μUTRN-corrected iPS-derived myogenic precursors in dKO mice. Serial cross-sections (total length of 1000 μm) of TA muscles collected from dKO mice that had been injected with PBS (contra-lateral leg) (a) or myogenic progenitors (b) were stained with antibodies to utrophin and several members of the dystrophin protein complex, including β-dystroglycan (β-DG), α1-syntrophin (α1-SYN) and neuronal nitric oxide synthase (nNOS) (red). These proteins were detected only in muscles transplanted with μUTRN-corrected myogenic precursors, in which they were found expressed in a contiguous manner across long sections of muscle fibre, as shown by the asterisks. Roman numbers within these images indicate the order of serial sections. PBS-injected dKO mice showed no signal for any of these proteins. 4,6-Diamidino-2-phenylindole (DAPI) is shown in blue. Scale bar, 50 μm. (c) Quantification of μUTRN+myofibers in these engrafted muscles (n=8). For each muscle, 3–4 representative cross-sections at 2-mm intervals were counted. For PBS control groups, we examined 20 random sections. Error bars represent s.d. Figure 2: Engraftment of μUTRN-corrected iPS-derived myogenic precursors in dKO mice. Serial cross-sections (total length of 1000 μm) of TA muscles collected from dKO mice that had been injected with PBS (contra-lateral leg) ( a ) or myogenic progenitors ( b ) were stained with antibodies to utrophin and several members of the dystrophin protein complex, including β-dystroglycan (β-DG), α1-syntrophin (α1-SYN) and neuronal nitric oxide synthase (nNOS) (red). These proteins were detected only in muscles transplanted with μUTRN-corrected myogenic precursors, in which they were found expressed in a contiguous manner across long sections of muscle fibre, as shown by the asterisks. Roman numbers within these images indicate the order of serial sections. PBS-injected dKO mice showed no signal for any of these proteins. 4,6-Diamidino-2-phenylindole (DAPI) is shown in blue. Scale bar, 50 μm. ( c ) Quantification of μUTRN + myofibers in these engrafted muscles ( n =8). For each muscle, 3–4 representative cross-sections at 2-mm intervals were counted. For PBS control groups, we examined 20 random sections. Error bars represent s.d. Full size image Engrafted corrected cells reestablish functional properties To investigate whether engraftment was accompanied by improvement in muscle function, we evaluated in a blinded manner the contractile properties of transplanted muscles compared with their contra-lateral leg controls. Engrafted muscles showed markedly superior isometric tetanic force ( Fig. 3a ) and increased absolute and specific force ( Fig. 3b , respectively) when compared with their respective contra-lateral PBS-injected TA muscles. No changes were observed in cross-sectional area (CSA) ( Supplementary Fig. S6c ) or weight ( Supplementary Fig. S6d ), as previously observed for ES-derived myogenic progenitors using this delivery route [12] . Data from the fatigue test showed no differences between transplanted and control groups ( Fig. 3d ), suggesting that levels of engraftment were not sufficient to restore this parameter. 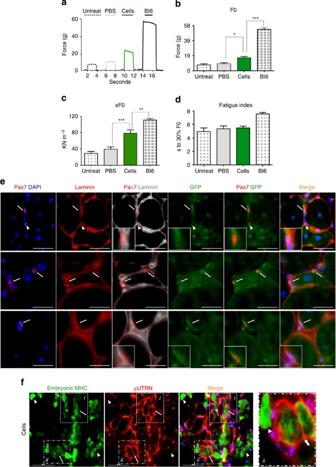Figure 3: Functional improvement and satellite cell engraftment of transplanted muscles. (a) Representative examples of isometric force tracking in TA muscles that had been injected with corrected cells or PBS (contra-lateral leg) (green and grey lines, respectively). For reference, untreated dKO and wild-type Bl6 mice controls are shown (dashed and black line, respectively). (b,c) Effect of cell transplantation on absolute (F0) and specific (sF0=F0 normalized to CSA) force, respectively. Error bars represent s.e.m. from a total of 13 transplanted mice. *P<0.05,**P<0.01 and***P<0.001. (d) Fatigue index: time for force to decline to 30% of maximal value during continuous stimulation of muscle at 150 Hz. (e)In situlocalization images show the presence of donor-derived satellite cells in engrafted dKO mice, as evidenced by the presence of Pax7+(red) and GFP+(green) cells under the basal lamina (indicated by arrows). Arrowheads denote endogenous Pax7+GFP−satellite cells. (f) Engrafted cells respond to CTX injury, giving rise to new myofibers as evidenced by the co-expression of μUTRN (red) and embryonic MHC (green). White arrows indicate μUTRN+/eMHC+donor-derived newly formed myofibers, and arrowheads point to μUTRN−/eMHC+host-derived newly formed myofibers. Scale bar, 50 μm. DAPI, 4,6-diamidino-2-phenylindole. Figure 3: Functional improvement and satellite cell engraftment of transplanted muscles. ( a ) Representative examples of isometric force tracking in TA muscles that had been injected with corrected cells or PBS (contra-lateral leg) (green and grey lines, respectively). For reference, untreated dKO and wild-type Bl6 mice controls are shown (dashed and black line, respectively). ( b , c ) Effect of cell transplantation on absolute (F0) and specific (sF0=F0 normalized to CSA) force, respectively. Error bars represent s.e.m. from a total of 13 transplanted mice. * P <0.05, ** P <0.01 and *** P <0.001. ( d ) Fatigue index: time for force to decline to 30% of maximal value during continuous stimulation of muscle at 150 Hz. ( e ) In situ localization images show the presence of donor-derived satellite cells in engrafted dKO mice, as evidenced by the presence of Pax7 + (red) and GFP + (green) cells under the basal lamina (indicated by arrows). Arrowheads denote endogenous Pax7 + GFP − satellite cells. ( f ) Engrafted cells respond to CTX injury, giving rise to new myofibers as evidenced by the co-expression of μUTRN (red) and embryonic MHC (green). White arrows indicate μUTRN + /eMHC + donor-derived newly formed myofibers, and arrowheads point to μUTRN − /eMHC + host-derived newly formed myofibers. Scale bar, 50 μm. DAPI, 4,6-diamidino-2-phenylindole. Full size image Transplanted cells seed the satellite cell compartment Next, we examined whether μUTRN-corrected myogenic precursors have the ability to seed the satellite cell compartment, and therefore to respond to injury ( Supplementary Fig. S6d ). To facilitate the detection of donor-derived satellite cells, corrected myogenic precursors were labelled with a lentiviral vector encoding GFP ( Supplementary Fig. S6d ). Three weeks following transplantation, we could clearly identify the presence of Pax7 + GFP + cells beneath the basal lamina ( Fig. 3e ), indicative of donor-derived satellite cells. This was confirmed by another experimental cohort, in which we promoted CTX injury in dKO mice that had been transplanted 3 weeks prior with μUTRN-corrected myogenic precursors (not labelled with GFP) ( Supplementary Fig. S6d ). One week after injury, we detected the presence of donor-derived newly formed corrected myofibers, as shown by the presence of μUTRN + /embryonic MHC + myofibers ( Fig. 3f ). Recipient-derived newly formed myofibers (μUTRN − /embryonic MHC + ) were found in transplanted mice ( Fig. 3f ) as well as in PBS-injected controls (contra-lateral leg; Supplementary Fig. S6e ), as expected. The donor-derived newly formed myotubes (eMHC + μUTRN + ; Fig. 3f ) could be derived from iPS-derived satellite cells (most likely because there are donor-derived satellite cells in engrafted muscles; Fig. 3e ), but could also form from a non-satellite myogenic precursor population that did not seed the satellite cell compartment and did not differentiate into myofibers. These results are of particular interest, as activation of corrected satellite cells could provide new μUTRN + myofibers during the progress of the muscular dystrophy, slowing the progression of the disease. Engrafted myofibers exhibit synaptic connections To address whether engrafted μUTRN + myofibers exhibited direct connection with motoneurons, we stained muscle sections with α-bungarotoxin (α-BTX). Our results clearly show the presence of nicotinic acetylcholine receptors at the neuromuscular junction of engrafted fibres ( Fig. 4 ). In wild-type mice, as expected, utrophin was detected solely at the neuromuscular junction, along with α-BTX ( Fig. 4c ), whereas in PBS-injected controls, only α-BTX was present ( Fig. 4b ). All together, these data suggest that μUTRN-corrected iPS-derived myogenic precursors integrate with the neuromuscular system. 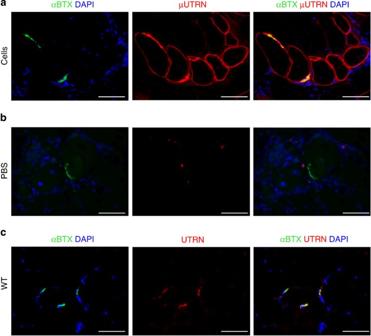Figure 4: Engrafted μUTRN+myofibers exhibit direct synaptic connections to motoneurons. Representative images show AChRs labelled with α-BTX in TA muscles that had been injected with corrected iPS-derived myogenic progenitors (a) or PBS (b). TA muscles from wild-type (WT) mice are also shown as a reference (c). Utrophin is indicated in red and α-BTX is shown in green. 4,6-Diamidino-2-phenylindole (DAPI) is shown in blue. Scale bar, 50 μm. Figure 4: Engrafted μUTRN + myofibers exhibit direct synaptic connections to motoneurons. Representative images show AChRs labelled with α-BTX in TA muscles that had been injected with corrected iPS-derived myogenic progenitors ( a ) or PBS ( b ). TA muscles from wild-type (WT) mice are also shown as a reference ( c ). Utrophin is indicated in red and α-BTX is shown in green. 4,6-Diamidino-2-phenylindole (DAPI) is shown in blue. Scale bar, 50 μm. Full size image Systemic cell transplantation in dKO mice Because reaching disparate muscle groups is critical when considering clinical application of cell therapy for DMD, we assessed engraftment levels following the systemic delivery of μUTRN-corrected iPS-derived myogenic precursors. Intravenous injection of these cell preparations resulted in distribution of donor-derived myofibers in several muscles, including TA, gastrocnemius lateralis and peroneal ( Fig. 5a–c ; Supplementary Table S1 ), of all the five mice that had been transplanted. In one of these mice, we were able to detected μUTRN-donor-derived myofibers in the diaphragm ( Supplementary Fig. S7a ). No utrophin signal was detected in any muscles from the PBS-injected mice ( Supplementary Figs S7b and S8 ; Supplementary Table S1 ). In this cohort of transplanted mice, no engraftment was observed in non-skeletal muscle tissues including heart, lung and liver ( Supplementary Fig. S9 ). This was also the case following the systemic injection of mouse ES cells, as previously reported [12] . 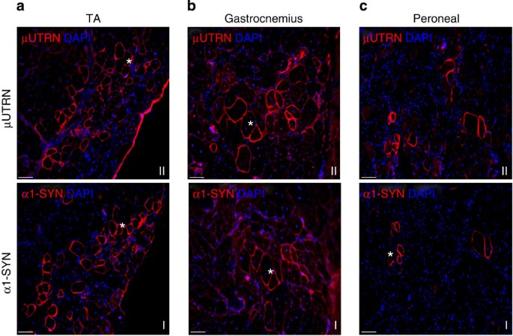Figure 5: Effective systemic delivery of μUTRN-corrected myogenic progenitors in dKO mice. Representative images reveal engraftment of TA (a), gastrocnemius lateralis (b) and peroneal (c) muscles of dKO mice that had received intravenous injection of corrected iPS-derived myogenic progenitors, as evidenced by staining with anti-utrophin and anti-α1-syntrophin (α1-SYN) antibodies. Roman numbers within these images indicate the order of serial sections. 4,6-Diamidino-2-phenylindole (DAPI) is shown in blue. Systemic delivery was performed in five dKO mice. Scale bar, 50 μm. Figure 5: Effective systemic delivery of μUTRN-corrected myogenic progenitors in dKO mice. Representative images reveal engraftment of TA ( a ), gastrocnemius lateralis ( b ) and peroneal ( c ) muscles of dKO mice that had received intravenous injection of corrected iPS-derived myogenic progenitors, as evidenced by staining with anti-utrophin and anti-α1-syntrophin (α1-SYN) antibodies. Roman numbers within these images indicate the order of serial sections. 4,6-Diamidino-2-phenylindole (DAPI) is shown in blue. Systemic delivery was performed in five dKO mice. Scale bar, 50 μm. Full size image Muscular dystrophies are a genetically and clinically heterogeneous group of neuromuscular diseases characterized by progressive skeletal muscle weakening that are commonly associated with paralysis and cardiopulmonary complications. Although no effective treatment is available at present, one attractive therapeutic approach is to use cell-based therapies to promote muscle regeneration. Skeletal muscle stem cells represent the ideal cell population to be utilized because transplantation of these cells results not only in efficient muscle regeneration but also in long-term maintenance through engraftment of the satellite stem cell pool; however, their therapeutic potential so far has been limited because of their scarcity in adult muscle, and the fact that in vitro expansion of these cells results in reduced engraftment ability [32] . Pluripotent stem cells are unique in terms of proliferation and differentiation potential, and therefore they represent an advantageous option for therapeutic application. We have demonstrated that following introduction of Pax3 or Pax7, transcription factors that have a critical role in skeletal myogenesis, both ES and control iPS cells give rise to myogenic progenitors endowed with the ability to promote muscle regeneration, to improve the contractility of engrafted muscles and to seed the satellite cell compartment following transplantation in dystrophic mice [11] , [12] , [13] , [14] , [33] . These encouraging data suggested that a similar positive outcome could potentially be achieved with patient-specific iPS cells. Our findings demonstrate for the first time proof-of-principle for the feasibility of combining iPS cell therapy in conjunction with genetic correction to treat muscular dystrophy. Although further refinements would be required before converting this proof-of-concept method to a clinical protocol, for example, non-integrating methods of delivering Pax3 or Pax7 and iPS reprogramming factors, as well as strategies to enhance engraftment following systemic delivery, these data clearly demonstrate that i) non-virally corrected iPS-derived myogenic precursors are able to engraft in vivo following local and systemic transplantation; ii) such expression restores components of the DGC and that engrafted myofibers exhibit neuromuscular synapses, iii) muscle strength can be significantly improved with this approach and iv) grafted μUTRN-corrected myogenic precursors seed the satellite cell compartment and contribute to muscle fibre repair, confirming that this strategy confers long-term expression of μUTRN protein. Generation of iPS cells and characterization TTF cultures were established by trypsin digestion of tail-tip biopsies taken from 3-week-old dKO mice. Fibroblasts were transduced with Oct3/4, Sox2 and Klf-4, and iPS clones were individually isolated as previously described [23] . Following initial expansion, iPS clones were characterized in vitro for SSEA-1 expression by flow cytometry (clone MC-480; eBioscience), as well as immunostaining for Nanog, Oct4 and SSEA-1 (R&D Systems). Alkaline phosphatase activity (Millipore) was also evaluated. iPS cells were subjected to karyotype analysis by G-banding. For the teratoma assay, one million cells suspended in 100 μl were injected subcutaneously into Rag2 −/− /IL2Rg −/− immunodeficient mice (Jackson Laboratory). One month after injection, teratoma was dissected and fixed with formalin. Tissues were sectioned and stained with hematoxylin and eosin. Cell culture ES and iPS cells were maintained as previously described [12] and differentiated, as follows: iPS cells were trypsinized and plated at 50,000 cells per cm 2 on a monolayer of mouse embryonic fibroblasts. At day 3, a single-cell suspension of pluripotent cells was obtained by pre-plating on gelatin in the presence of EB medium for 1 h. These cells were then cultured as cell suspension at 10,000 cells per ml of EB medium and incubated on a slowly swirling table rotator at 70 r.p.m. (set up inside of the tissue culture incubator). At day 3 of EB differentiation, 0.8 μg ml −1 of doxycycline was added to the medium to induce Pax3. At day 5, EBs were trypsinized and stained for PDGFαR and Flk-1. Sorted cells were plated onto fresh gelatin-coated flasks at 100,000 cells per cm 2 in the presence of proliferation myogenic medium, which consisted of IMDM, 15% FBS, 1% chicken embryo extract, 10% horse serum, supplemented with 1 μg ml −1 of doxycycline and 5 ng ml −1 of bFGF. For terminal differentiation, medium was switched to low glucose DMEM, and 5% horse serum (no dox or bFGF). Plasmids and generation of iPax3-μUTRN iPS cells We developed a T2-inverted terminal repeat Tn vector (pKt2/μUTRN) carrying a 7.3-kb engineered transgene containing μUTRN and an iresGFP reporter, which allows for the selection of μUTRN-corrected iPS cells. The whole transgene is flanked by the terminal inverted repeats (IR/DR), each of which contains two binding sites for the transposase itself (DR). Flag-μUTRN was engineered by recombinant PCR using the same primers described previously for TAT-μUtr [20] , except that Bam HI and Bst BI were used to cut pFastBac Flag-Utr [34] to reintroduce the recombined Flag-μUTRN into pFastBac1. Pfu Ultra polymerase was used for all PCR, and constructs were confirmed by DNA sequence analysis. This Flag-μUTRN construct was cloned into the pORF5-mcs vector (Invitrogen), and then a blunted EcoR I- Cla I iresGFP fragment was cloned into the blunted Nde I site of the pORF5-μUTRN vector. Finally, the blunted Pac I- Asi sI transgene containing promoter-μUTRN-iresGFP-pA was cloned into pKT2 vector. For transposase, we used pCMV-SB100X (generously provided by Zoltan Ivics from Max Delbruck Center for Molecular Medicine, Berlin), which yields high levels of Tn integration [28] . The inducible iPax3 vector was generated by cloning the full-length Pax3 coding sequence from Open Biosystems (clone MMM1013-9201572) into pSAM2-iresCherry vector. Plasmids were prepared using an Endofree Midiprep kit (Nucleobond). For SB transposase-mediated integration of μUTRN Tn, 3 × 10 5 iPS cells were nucleofected with 1 μg of pCMV-SB100 and 5 μg of μUTRN-pKT2 using Nucleofector 96-well Shuttle (program CG-108) (Lonza). Corrected iPS cells were purified based on sorting for GFP + cells. The doxycycline tet-responsive Pax3 cells were generated by transducing iPS cells with both iPax3/ires-mCherry and rtTA lentiviral constructs. Stable iPax3-iPS cells were purified based on mCherry expression by FACS. RT–PCR and western blot analyses Real-time PCR for pluripotency and muscle-specific genes was performed using probe sets from Applied Biosystems. In the case of μUTRN, the gene expression assay was customized by Applied Biosystems ( Supplementary Table S2 ). For western blot, cell lysates were prepared using X1 RIPA buffer (Thermo Scientific) in combination with Complete Protease Inhibitor Cocktail (Roche) and PhosSTOP (Roche). A total of 50 μg of protein lysates was loaded in each lane, resolved in SDS–PAGE and transferred to membranes (Immobilon-P; Millipore), which were incubated overnight at 4 °C with primary antibodies: utrophin mAb 8A4 (1:50; Santa Cruz Biotechnology), anti-FLAG mAb M2 (1:1,000; Sigma), Actin (1:3,000; GenScript), Pax3 (1:1,000; R&D Systems) and GAPDH (1:3,000; Abcam). After incubation with horseradish peroxidase-conjugated secondary antibodies (1:10,000; Amersham), membranes were incubated with Chemiluminescent Substrate (Thermo Scientific) and exposed to film. FACS analysis EB-derived cells were collected with trypsin (2 min at 37 °C), washed in staining buffer (PBS, 2% FBS), suspended in the same buffer containing 0.25 μg per 10 6 cells of Fc block (eBioscience) and incubated on ice for 5 min. Cells were then incubated on ice for 30 min with specific antibody (1 μg per 10 6 cells). For PDGFαR and Flk-1, phycoerythrin- and antigen-presenting cell (APC)-conjugated antibodies, respectively, were used (eBioscience). For the characterization of myogenic precursors, cells were collected using dissociation buffer (10 min at 37 °C). We used the following antibodies: anti-M-cadherin (clone 5; Pharmingen), APC-conjugated anti-CXCR4 (BD Biosciences), anti-VCAM1 (eBioscience) and anti-CD56 (Miltenyi), as well as phycoerythrin-conjugated anti-Syndecan4 (Pharmingen). For secondary staining in the case of M-cadherin, we used APC-conjugated goat anti-mouse Ig (Pharmingen). Stained cells were analysed and sorted on a FACS Aria (Becton Dickinson). Immunofluorescence of cultured cells and tissue sections Immunofluorescence staining of μUTRN and representative components of the DGC was performed on tissue cryosections. TA muscles were embedded in Tissue-Tek OCT compound, and immediately frozen in isopentane cooled in liquid nitrogen. Cut tissues (10–12 μm) were blocked for 30 min in 4% BSA and 0.05% Tween-20, followed by overnight incubation with specific primary antibody in PBS containing 2% goat serum. After three PBS washes, sections were incubated for 45 min with secondary antibody. All primary antibodies were made in rabbit, as follows: rabbit anti-utrophin polyclonal antibody (1:400); rabbit anti-α1-Syntrophyn (1:200) (kindly provided by Stan Froehner, University of Washington); rabbit anti-β-dystroglycan (1:400) (H-242 sc-28535; Santa Cruz Biotechnology); rabbit anti-nNOS (1:100; Sigma); mouse anti-Pax7 (1:250; MAB 1675; R&D System); rabbit anti-Laminin (1:400; Sigma), chicken anti-GFP (1:250; ab1390; Abcam), α-BTX (1:500; Invitrogen) and anti-embryonic MyHC (1:20; F1.652; Developmental Studies Hybridoma Bank). For Pax7 staining, MOM kit (Vector Laboratory) was used following the manufacturer’s instruction. For secondary staining, goat Alexa-555 anti-rabbit or mouse, Alexa-488 anti-rabbit or mouse, Alexa-647 anti-rabbit and Alexa-488 anti-chicken (1:1,000) were used (Molecular Probes). Control tissues were processed simultaneously in the same manner. For in vitro cultures, cells were maintained on gelatin-coated plates and processed as described above. For nuclear staining, cells were first fixed for 10 min at −20 °C in 100% ice-cold methanol, washed twice in PBS and incubated for 10 min with 0.3% Triton X-100 in PBS. The following primary antibodies were used: anti-Pax3 (1:100; R&D Systems), anti-Myf5 (1:100; C-20; Santa Cruz Biotechnology), anti-MyoD (1:100; Pharmingen) and anti-MyHC (1:50; M20; Developmental Studies Hybridoma Bank). Alexa fluor 555 and 488 goat anti-rabbit (Molecular Probes) were used for secondary staining. 4,6-Diamidino-2-phenylindole (Sigma) was used to counter-stain nuclei. Mice and transplantation studies Animal experiments were carried out according to the protocols approved by the University of Minnesota Institutional Animal Care and Use Committee. Dystrophin/utrophin-deficient (mdx ;utrn −/− ) mice (total of 23 dKO mice) were derived and genotyped as previously described [18] . One day before cell transplantation (for both intramuscular or intravenous injections), mice were started on an daily immunosuppression regimen (FK-506, also known as Tacrolimus) for the duration of the experiment, as previously described [12] . Myogenic progenitor cells were collected using dissociation buffer (10 min at 37 °C), and then injected directly into the left TA muscle (10 6 cells per 10 μl PBS) or alternatively, through the tail vein for systemic delivery (0.8 × 10 6 cells per 150 μl DMEM 10% FBS). Control mice received the same volume of PBS. Mice were injured with 50 μl of CTX (10 μM; Sigma) only in experiments aimed to investigate the capacity of engrafted satellite cells to give rise to myofibers expressing the truncated utrophin. Muscle preparation for mechanical studies For the measurement of contractile properties, mice were anaesthetized with avertin (250 mg kg −1 intraperitoneal), and intact TA muscles were dissected and placed in an experimental organ bath as previously described in detail [12] . Muscles were stimulated by an electric field generated between two platinum electrodes placed longitudinally on either side of the muscle (square wave pulses 25 V, 0.2 ms in duration, 150 Hz). Muscles were adjusted to the optimum length ( Lo ) for the development of isometric twitch force, and a 5-min recovery period was allowed between stimulations. Optimal muscle length ( Lo ) and stimulation voltage (25 V) were determined from micromanipulation of muscle length and a series of twitch contractions that produced maximum isometric twitch force. For measuring fatigue time, muscles were stimulated for 1 min, and the time for force to decline to 30% of Fo was measured. In brief, after determination of optimal muscle length ( Lo ) and measurement of maximum isometric tetanic force, total muscle CSA was calculated by dividing muscle mass (mg) by the product of muscle length (mm) and 1.06 mg mm −3 , the density of mammalian skeletal muscle. Specific force was determined by normalizing maximum isometric tetanic force to CSA. Statistical analysis Differences between samples were assessed by using one-way analysis of variance. All data are presented as mean±s.e.m. How to cite this article: Filareto, A. et al . An ex vivo gene therapy approach to treat muscular dystrophy using inducible pluripotent stem cells. Nat. Commun. 4:1549 doi: 10.1038/ncomms2550 (2013).